Manipulation of B-cell responses with histone deacetylase inhibitors Histone deacetylase inhibitors (HDACi) are approved for treating certain haematological malignancies, however, recent evidence also illustrates they are modulators of the immune system. In experimental models, HDACi are particularly potent against malignancies originating from the B-lymphocyte lineage. Here we examine the ability of this class of compounds to modify both protective and autoimmune antibody responses. In vitro , HDACi affect B-cell proliferation, survival and differentiation in an HDAC-class-dependent manner. Strikingly, treatment of lupus-prone Mrl /lpr mice with the HDACi panobinostat significantly reduces autoreactive plasma-cell numbers, autoantibodies and nephritis, while other immune parameters remain largely unaffected. Immunized control mice treated with panobinostat or the clinically approved HDACi vorinostat have significantly impaired primary antibody responses, but these treatments surprisingly spare circulating memory B cells. These studies indicate that panobinostat is a potential therapy for B-cell-driven autoimmune conditions and HDACi do not induce major long-term detrimental effects on B-cell memory. B cells are responsible for the production of soluble antibody that defends the host against invading foreign pathogens. B cells are typically activated by binding of foreign antigen to the B-cell receptor (BCR), which induces B-cell activation and a cascade of interactions with immune helper cells and cytokines. After activation, B cells either (a) form short-lived extrafollicular plasmablasts that are critical for early protective immunity or (b) enter specialized germinal centres where they undergo extensive proliferation and produce novel immunoglobulin molecules via somatic hypermutation. This process yields both plasma cells that secrete high affinity antibodies and long-lived memory B cells that confer long-term protection from re-challenge with antigen [1] , [2] , [3] , [4] . Major genetic abnormalities such as chromosomal translocations, or subtle disruption of proliferation, programmed cell death or differentiation at any stage of an antibody response can have drastic consequences on human health. For example, constitutive expression of proto-oncogenes driven by chromosomal translocations with immunoglobulin gene loci can lead to the development of B-cell neoplasms such as follicular, Burkitt or diffuse large B-cell lymphoma [5] , [6] , [7] , [8] . Alternatively, the failure to eliminate or control proliferation of self-reactive B cells can trigger autoimmunity [9] , [10] . This is best illustrated in B-cell-mediated autoimmune conditions such as systemic lupus erythematosus (SLE, ‘lupus’), which results from an accumulation of self-reactive antibody-secreting B cells and manifests with multi-organ pathologies including vasculitis and glomerulonephritis [11] . As B-cell autoimmune conditions arise from a number of diverse molecular or genetic aberrations that are indistinguishable at disease presentation [11] , targeting pathogenic autoantibody-secreting cell populations while preserving protective immune subsets is of utmost importance. Similarly, development of novel therapies that allow aggressive targeting of B-cell malignancies without compromising protective immunity remains a clinical goal. Accumulating evidence has demonstrated that epigenetic changes play a key role in shaping gene expression profiles of differentiating lymphocytes [12] , [13] . Similarly, mice deficient in histone deacetylase (HDAC) enzymes 1 and 2 have disrupted B-cell development, survival and activation [14] , [15] , [16] . Therefore, pharmacological targeting of epigenetic enzymes such as HDACs arises as a potential method for manipulating antibody responses. HDAC inhibitors (HDACi) are a class of compounds capable of remodelling chromatin and altering gene expression through the induction of histone hyperacetylation. In addition, HDACi can affect the acetylation status of non-histone proteins [17] . Treatment of tumour cells with HDACi can affect apoptosis, cell cycle arrest and differentiation. Moreover, these agents can suppress tumour angiogenesis and enhance anti-tumour immunity [17] . The HDACi vorinostat (Zolinza) and romidepsin (Istodax) are FDA approved for the treatment of cutaneous T-cell lymphoma and trials are ongoing to determine the effectiveness of these drugs in other haematological diseases [18] . In addition, in experimental animal models, both B-cell and plasma-cell malignancies are sensitive to HDACi treatment [19] , [20] . The wealth of experimental data on the effect of HDACi on cancer cells including haematological malignancies, has progressed these compounds into the clinic. Interestingly, emerging data illustrate that HDACi can also modify lymphocyte subsets such as T cells [21] , [22] , T regs [23] and B cells [24] , [25] . The potential to modify autoantibody responses is highlighted by data illustrating experimental HDACi such as Trichostatin A (which has not progressed into the clinic) can reduce antibody production in cell lines in vitro [24] while vorinostat treatment of MRL /lpr mice dampens immune cytokines such as IL-2, IFN-γ, IL-6 and IL-10 (ref. 25 ). Thus, HDACi have been proposed as potential therapeutic agents for treatment of B-cell-mediated autoimmune diseases [25] , [26] , [27] , [28] . However, the direct functional effect of HDACi on the protective B-cell response and consequence for cancer patients undergoing HDACi therapy, how specific classes of HDACi regulate components of the antibody response, and analysis of newly emerging HDACi such as panobinostat has not yet been determined. Recently, quantitative systems have emerged as a powerful tool for dissecting components that contribute to lymphocyte responses in vitro [29] , [30] , [31] , [32] . The aim of this study was to dissect how these compounds affected the separate components of the protective antibody response and shed light on the possible immunological consequences for cancer patients post HDACi therapy. In addition, we wanted to determine whether emerging HDACi such as panobinostat have potential as therapies for B-cell-dependent autoimmune conditions. Here, we demonstrate that HDACi are capable of manipulating in vitro and in vivo antibody responses in a HDAC-class-dependent manner. Importantly, the HDACi panobinostat is capable of targeting autoreactive B-cell populations while sparing long-term memory cells and other components of the immune system. These findings have exciting ramifications for the treatment of B-cell-mediated autoimmune disease. In vitro survival and proliferation are HDACi class-dependent Initially, we investigated the effect of vorinostat and panobinostat (that target class I, II and IV HDACs) and the class-I-selective HDACi romidepsin on B-cell responses in vitro . To dissect the effects of specific HDACi on the antibody response in vitro , we performed a quantitative analysis of B-cell survival, proliferation and division. Highly purified naive B cells were isolated from C57BL/6 mice and labelled with CFSE to track cell division. To isolate the effect of HDACi solely on the B-cell compartment, we used soluble stimuli to mimic T-cell help, which removes the variable of intrinsic alterations to T-cell function that provide help. We chose the soluble crosslinking anti-CD40 antibody 1c10 because when used in the presence of saturating IL-4, it induces typical proliferation, differentiation and isotype switching as membrane-bound CD40L [31] , [33] . B cells were cultured in varying concentrations of HDACi and daily quantitative measurements of viability, cell numbers and division progression determined by flow cytometry [29] , [31] . In cultures treated with vorinostat and panobinostat, cell viability as a proportion of total ( Fig. 1a ) and cell number ( Fig. 1b and Supplementary Fig. 1a ) were reduced after 24 h in a dose-dependent manner. Similar results were observed with romidepsin, although apoptosis was more apparent 48 h after treatment ( Fig. 1a,b and Supplementary Fig. 1a ). Concomitant with the effects on cell viability, vorinostat and panobinostat had a significant impact on the ability of B cells to progress through division ( Fig. 1c ). The combined effect on survival and division resulted in a significant decrease in the number of B cells per division ( Fig. 1d ) and total cell number ( Fig. 1b ). In contrast, after romidepsin treatment, remaining viable B cells still progressed through an equivalent number of divisions as untreated cultures ( Fig. 1c,d ). 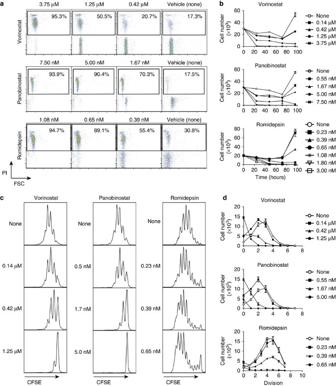Figure 1: HDACi modulate T-cell-dependent B-cell responsesin vitro. CFSE-labelled B cells were stimulated with αCD40+IL-4 in the presence of the indicated concentrations of class I/II HDACi and the response measured over four days. (a) Viability of HDACi-treated B cells was determined by exclusion of propidium iodide using flow cytometry, and (b) numbers of live cells were quantified by measurement relative to a known number of calibration beads. Ina, vorinostat and panobinostat responses are shown after 24 h while romidepsin responses are shown after 48 h. CFSE profiles of HDACi-treated B cells were used to determine progression through cell division. (c) CFSE profiles for day 3 are shown and (d) cell numbers in each division are quantified as described in Methods. Data inaandcare representative plots from triplicate samples. Data inbanddare mean±s.e.m. of triplicate samples. All data are representative from three independent experiments. Figure 1: HDACi modulate T-cell-dependent B-cell responses in vitro . CFSE-labelled B cells were stimulated with αCD40+IL-4 in the presence of the indicated concentrations of class I/II HDACi and the response measured over four days. ( a ) Viability of HDACi-treated B cells was determined by exclusion of propidium iodide using flow cytometry, and ( b ) numbers of live cells were quantified by measurement relative to a known number of calibration beads. In a , vorinostat and panobinostat responses are shown after 24 h while romidepsin responses are shown after 48 h. CFSE profiles of HDACi-treated B cells were used to determine progression through cell division. ( c ) CFSE profiles for day 3 are shown and ( d ) cell numbers in each division are quantified as described in Methods. Data in a and c are representative plots from triplicate samples. Data in b and d are mean±s.e.m. of triplicate samples. All data are representative from three independent experiments. Full size image It has previously been hypothesized that HDACi control TNF super family pathways [34] including CD40 signalling. Furthermore, T-cell-dependent and -independent signalling has been shown to regulate B-cell responses in a distinct manner [31] . Therefore, to determine whether the effects of HDACi on B-cell responses were able to regulate a broad range of B-cell responses, we repeated our previous assays in the context of T-cell-independent stimulation through TLR-4 using lipopolysaccharide (LPS). Consistent with assays shown in Fig. 1 , vorinostat, panobinostat and romidepsin all affected the survival of LPS-stimulated B cells ( Fig. 2a,b and Supplementary Fig. 1b ). Similarly, division progression was delayed by vorinostat and panobinostat, while romidepsin had little effect ( Fig. 2c,d ). Together, these results demonstrate that some classes of HDACi broadly affect B-cell survival and proliferation. An important distinction, however, was that the class-I specific inhibitor romidepsin did not affect B-cell proliferation in the same manner as more broadly acting HDACi. Hence, romidepsin-treated cultures still progressed through an equivalent number of cell divisions as determined by the mean division number ( Supplementary Fig. 2 ). Importantly panobinostat, which has not previously been extensively studied in the context of B-cell function, is a potent modifier of antibody responses to both T-dependent and -independent stimulation. 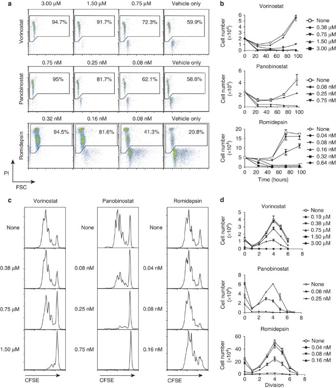Figure 2: HDACi modulate T-cell-independent B-cell responsesin vitro. CFSE labelled B cells were stimulated with LPS in the presence of the indicated concentrations of class I/II HDACi and their response measured over 4 days. (a) Viability of B cells was determined by exclusion of propidium iodide using flow cytometry, and (b) numbers of live cells were quantified by measurement relative to a known number of calibration beads. Ina, vorinostat and panobinostat responses are shown after 24 h while romidepsin responses are shown after 48 h. CFSE profiles of HDACi-treated B cells were used to determine progression through cell division. (c) Division profiles for day 3 are shown and (d) cell numbers in each division are quantified. Data inaandcare representative plots from triplicate samples. Data inbanddare mean±s.e.m. of triplicate samples. All data are representative from three independent experiments. Figure 2: HDACi modulate T-cell-independent B-cell responses in vitro. CFSE labelled B cells were stimulated with LPS in the presence of the indicated concentrations of class I/II HDACi and their response measured over 4 days. ( a ) Viability of B cells was determined by exclusion of propidium iodide using flow cytometry, and ( b ) numbers of live cells were quantified by measurement relative to a known number of calibration beads. In a , vorinostat and panobinostat responses are shown after 24 h while romidepsin responses are shown after 48 h. CFSE profiles of HDACi-treated B cells were used to determine progression through cell division. ( c ) Division profiles for day 3 are shown and ( d ) cell numbers in each division are quantified. Data in a and c are representative plots from triplicate samples. Data in b and d are mean±s.e.m. of triplicate samples. All data are representative from three independent experiments. Full size image In vitro B-cell differentiation is HDACi class-dependent In response to T-cell-dependent stimulation, B cells may differentiate into effector, CD138 + antibody-secreting cells (ASC). As treatment with HDACi significantly reduces cell survival and proliferation, measurement of immunoglobulin levels in supernatant does not accurately represent the effect on the differentiation compartment. Therefore, we quantified the generation of CD138 + B cells relative to division in the presence of HDACi to remove this bias. As seen previously ( Figs 1 and 2 ), vorinostat and panobinostat inhibited the progression of B cells through division in a dose-dependent manner and led to a substantial decrease in the overall proportion of CD138 + cells ( Fig. 3a ). When the effect of cell division was removed, we noted a reduction in the proportion of ASCs on a per-division basis ( Fig. 3b ). Interestingly, the small proportion of B cells still capable of progressing through division in the presence of high concentrations of romidepsin ( Fig. 3a ) were still capable of differentiating into ASC with only a slight difference observed in the proportion of ASC generated per division ( Fig. 3b ). These results were consistent with proliferation data and demonstrated that pan-HDACi significantly affects multiple facets of the antibody response while the class-I-selective HDACi romidepsin predominantly affected B-cell survival. 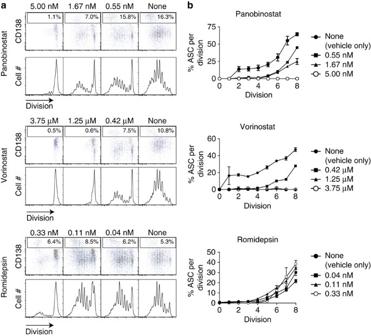Figure 3: HDACi modulate B-cell differentiation in a class-dependent manner. CFSE-labelled B cells were stimulated with αCD40+IL-4, treated with the indicated concentrations of HDACi and differentiation to ASC measured. After 4 days in culture, (a) differentiation to ASC was determined by expression of CD138 in relation to cell division and (b) quantified as proportion of ASC per division. Data inaare representative plots of triplicate samples. Data inbare mean±s.e.m. of triplicate samples. All data are representative from three independent experiments. Figure 3: HDACi modulate B-cell differentiation in a class-dependent manner. CFSE-labelled B cells were stimulated with αCD40+IL-4, treated with the indicated concentrations of HDACi and differentiation to ASC measured. After 4 days in culture, ( a ) differentiation to ASC was determined by expression of CD138 in relation to cell division and ( b ) quantified as proportion of ASC per division. Data in a are representative plots of triplicate samples. Data in b are mean±s.e.m. of triplicate samples. All data are representative from three independent experiments. Full size image We reasoned that the ability of panobinostat and vorinostat to broadly target B-cell growth, differentiation and survival made them the best potential candidates to target autoreactive B cells in vivo . In addition, the ability of panobinostat to significantly affect B-cell responses at low nanomolar concentrations makes it an attractive potential therapeutic to test in vivo for altering B-cell responses. However, vorinostat has been suggested to regulate CD3-primed CD8 T-cell responses in vivo [35] , and to cause significant CD8 + T-cell immunosuppression in comparison with panobinostat [36] . Therefore, we analysed the response of CD8 + T cells to HDACi treatment in vitro . CFSE-labelled CD8 + T cells were stimulated in vitro in the presence of vorinostat and panobinostat and their response measured. Although vorinostat affected T-cell survival and proliferation at the concentrations previously used to modify B-cell responses, panobinostat treatment did not, even at doses that induced significant change in B cells ( Supplementary Fig. 3 ). This highlighted that B cells are more sensitive than CD8 + T cells and furthermore, this response is HDACi specific. Although higher concentrations of panobinostat might elicit some effect on T-cell function, these results suggest at low doses, panobinostat could be used effectively to preferentially target B-cell responses in vivo and leave the T-cell compartment less affected. Panobinostat reduces disease burden in SLE mouse models We next investigated whether panobinostat could be used to eliminate auto-antibody-producing plasma cells using the MRL /lpr mouse autoimmunity model that exhibits systemic immune activation and auto-antibody production [37] . Groups of MRL /lpr mice 12–13 weeks old were treated daily with a reduced dose of panobinostat compared with preclinical studies with multiple myeloma [38] . Mice were monitored daily by a researcher masked to treatment groups and consistent with the recent panobinostat clinical trials [39] , no adverse effects were noted on the general well-being of mice. Furthermore, no significant changes were observed in the weights of animals throughout the treatment window ( Supplementary Fig. 4 ). Circulating B cells and plasma cells were identified and quantified on the basis of expression of B220 and CD138 ( Fig. 4a ). After 14 days, there was a dramatic reduction in the number of total B220 + CD19 + B cells and CD138 + B220 + ASC in the blood of panobinostat-treated mice ( Fig. 4b ), which was sustained over 29 days of treatment ( Fig. 4b ). The effect on plasma-cell numbers resulted in the significant reduction of antinuclear antibody titres in the serum as determined by measuring levels of antibody reactive against pooled dsDNA, histones, SSA/Ro, SSB/La and anti-Smith proteins ( Fig. 4c ). Single antigen specificity of antibodies were further dissected using an assay for extractable nuclear antigens (ENA) analysis modified for mouse serum. This analysis demonstrated a significant reduction in 5 of the 14 auto-antigens tested in panobinostat-treated mice ( Supplementary Fig. 5 ), including anti-dsDNA and anti-Sm, two autoantibodies virtually pathognomonic for SLE in humans. 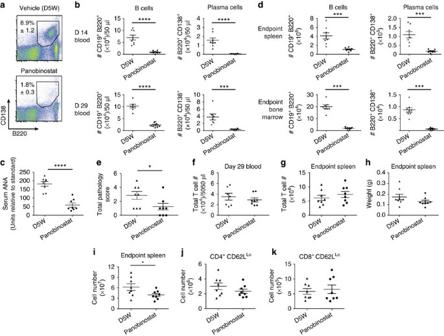Figure 4: Panobinostat treatment reduces autoimmune disease severity in MRL/lprmice. (a) Flow cytometric identification of plasma cells in the spleen of vehicle or panobinostat-treated MRL/lprmice based on expression of B220 and CD138. (b) Recirculating B cells (CD19+, B220+) and plasma cells (B220+, CD138+) were quantified in peripheral blood of vehicle or panobinostat-treated mice after 14 and 29 days by flow cytometry as shown ina. (c) Pooled antinuclear antibodies (ANA) in the serum of mice were measured after 29 days of panobinostat treatment. (d) After 42 days of panobinostat treatment, cohorts of mice were euthanized and B cells (CD19+, B220+) and plasma cells (B220+, CD138+) quantified in spleen and bone marrow. (e) After 42 days of treatment, haematoxylin and eosin sections of kidneys in treated and untreated cohorts were analysed as described in Methods and assigned a pathology score on the basis of disease severity. (f) T cells were identified on the basis of expression of CD4 or CD8 and quantified in peripheral blood after 29 days of treatment. After 42 days of panobinostat treatment, cohorts of mice were euthanized and assessed for (g) total T-cell number (CD4+and CD8+), (h) spleen weight and (i) total cell numbers. The numbers of activated (j) CD4+CD62Lloand (k) CD8+CD62LloT cells in spleen were also determined;n=8 for all groups. Significance of differences were determined using two-tailed unpairedt-tests. *P≤0.05, ***P≤0.001, ****P≤0.0001. Figure 4: Panobinostat treatment reduces autoimmune disease severity in MRL /lpr mice. ( a ) Flow cytometric identification of plasma cells in the spleen of vehicle or panobinostat-treated MRL /lpr mice based on expression of B220 and CD138. ( b ) Recirculating B cells (CD19 + , B220 + ) and plasma cells (B220 + , CD138 + ) were quantified in peripheral blood of vehicle or panobinostat-treated mice after 14 and 29 days by flow cytometry as shown in a . ( c ) Pooled antinuclear antibodies (ANA) in the serum of mice were measured after 29 days of panobinostat treatment. ( d ) After 42 days of panobinostat treatment, cohorts of mice were euthanized and B cells (CD19 + , B220 + ) and plasma cells (B220 + , CD138 + ) quantified in spleen and bone marrow. ( e ) After 42 days of treatment, haematoxylin and eosin sections of kidneys in treated and untreated cohorts were analysed as described in Methods and assigned a pathology score on the basis of disease severity. ( f ) T cells were identified on the basis of expression of CD4 or CD8 and quantified in peripheral blood after 29 days of treatment. After 42 days of panobinostat treatment, cohorts of mice were euthanized and assessed for ( g ) total T-cell number (CD4 + and CD8 + ), ( h ) spleen weight and ( i ) total cell numbers. The numbers of activated ( j ) CD4 + CD62L lo and ( k ) CD8 + CD62L lo T cells in spleen were also determined; n =8 for all groups. Significance of differences were determined using two-tailed unpaired t -tests. * P ≤0.05, *** P ≤0.001, **** P ≤0.0001. Full size image After 42 days panobinostat treatment, mice were euthanized and B-cell populations in spleen and bone marrow quantified. There was a significant reduction in naive B-cell and plasma-cell populations of treated mice, highlighting that B cells in peripheral lymphoid organs were sensitive to panobinostat ( Fig. 4d ). Consistent with the reduction in plasma-cell numbers and autoantibodies in serum, typical renal pathology of MRL /lpr mice including histological evidence of glomerulonephritis and interstitial nephritis was markedly and significantly reduced by panobinostat treatment ( Fig. 4e and Supplementary Fig. 6 ). As autoimmunity in MRL /lpr mice has been proposed to result from systematic activation of the lymphocyte compartment [37] , we also measured the effect of panobinostat treatment on T-cell numbers. In stark contrast to B-cell populations, and consistent with our in vitro data ( Supplementary Fig. 3 ), total T-cell numbers in the blood ( Fig. 4f ) and spleen ( Fig. 4g ) were unaffected by panobinostat treatment. Although we observed a reduction in total cell numbers, spleen weights in treated and untreated mice were similar ( Fig. 4h,i ) suggesting that the rapid loss of B-cell populations was not reflected across all haematopoietic lineages and blood cell populations. In addition, we detected no change in activated CD62L lo CD4 + and CD8 + T-cell populations in panobinostat-treated mice ( Fig. 4j,k ). Collectively, this suggests that the B-cell compartment is more sensitive to panobinostat than other blood cell lineages. To demonstrate the therapeutic effects of HDACi in a different model of autoimmunity, we tested for efficacy in mice with a loss of function mutation in Lyn, a Src kinase family member and downstream regulator of BCR signalling [40] that also accumulate high levels of pathogenic autoantibodies [41] , [42] , [43] . In this model, panobinostat caused a dramatic reduction in autoantibody levels ( Supplementary Fig. 7a and b ). Although antibody-secreting plasma cells are not detectable in peripheral blood of Lyn −/− mice, we noted that naive B-cell populations were particularly sensitive while T-cell numbers were maintained in panobinostat-treated mice ( Supplementary Fig. 7c and d ). Collectively, these data suggest that panobinostat may have broad therapeutic applicability for the treatment of B-cell-driven autoimmune disease, regardless of the molecular events that underpin the development of autoreactive plasma cells. Moreover, T-cell populations were again maintained in panobinostat-treated mice suggesting that B-lineage cells, including plasma cells responsible for autoimmune pathology, were more sensitive to the effects of panobinostat than other blood lineage cells. HDACi inhibit primary germinal center responses As HDACi are used clinically for the treatment of haematological malignancies, our results suggest that it is important to understand their effects on the production of protective antibody responses. We measured the effect of panobinostat in C57BL/6 mice immunized with the T-cell-dependent antigen, 4-hydroxy-3-nitrophenyl acetyl (NP) coupled to carrier protein keyhole limpet haemocyanin (NP–KLH). Mice received alum-adjuvanted NP–KLH intraperitoneally, and 5 days later were commenced either on vehicle or panobinostat for 7 days [44] . Fourteen days post immunization, spleens were harvested from mice treated with vehicle or panobinostat and the number of NP-responsive B cells quantified via flow cytometry to determine any overall effect on the protective immune response. Corresponding samples from quantified spleens were taken for histological analysis to determine changes in the organization of the germinal centre structure. The primary antibody response was significantly impaired in panobinostat-treated mice with the proportion and number of NP + IgG1 + -reactive B cells significantly reduced overall and within the GC compartment ( Fig. 5a–d ). Although fractionation of NP-responsive B cells into GC and memory cells based on CD38 expression ( Fig. 5c and Supplementary Fig. 8a ) revealed a bias towards the memory lineage in panobinostat-treated mice, this was due to the selective loss of GC B cells. Given the significant quantitative difference in GC B cells, we also investigated structural changes by immunofluorescence. Consistent with flow cytometry data, GC were less frequent in panobinostat-treated spleens ( Supplementary Fig. 9 ). Of the GC that were found, structural analysis by immunofluorescence revealed significant disruption of both the IgD + B-cell follicles and the GL-7 + GC, consistent with quantification by flow cytometry ( Fig. 5e and Supplementary Fig. 9 ). Given the striking effect of panobinostat treatment on GC formation in NP–KLH-immunized mice, we investigated whether panobinostat had a similar effect on GC in autoimmune MRL/ lpr mice. As GC are present in MRL/lpr mice before 2 months of age [45] , groups of MRL /lpr mice 7 weeks old were treated daily with panobinostat for 2 weeks and the effect on GC in the spleens determined by immunohistochemistry. Consistent with NP–KLH-immunized mice, MRL/ lpr mice treated with panobinostat had a significant reduction in both the number and percentage of GL-7 + GCs ( Supplementary Fig. 10 ). 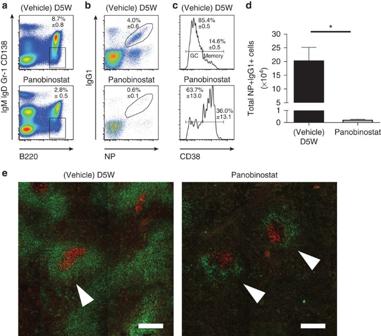Figure 5: Panobinostat inhibits primary antibody responses. Analysis of C57BL/6 mice 14 days after immunization with NP–KLH in alum and treatment with panobinostat. (a) Flow cytometric identification of isotype-switched splenic B cells (GR-1−, CD138−, IgM−, IgD−, B220+) and (b) gated, isotype-switched B cells analysed for reactivity against NP antigen (NP+, IgG1+). (c) NP+IgG1+B cells were further fractionated into germinal center (GC) and memory compartments on the basis of CD38 expression. (d) Absolute numbers of NP+IgG1+B cells per spleen. (e) Frozen sections of spleens 14 days post immunization stained with IgD (green) to identify B-cell follicles and GL-7 (red) to identify GC. Scale bars, 400 μm. White arrows indicate GC structures. Data are mean±s.e.m. of five mice per group. Data are representative of three independent experiments. Significance of differences were determined using two-tailed unpairedt-tests. *P<0.05. Figure 5: Panobinostat inhibits primary antibody responses. Analysis of C57BL/6 mice 14 days after immunization with NP–KLH in alum and treatment with panobinostat. ( a ) Flow cytometric identification of isotype-switched splenic B cells (GR-1 − , CD138 − , IgM − , IgD − , B220 + ) and ( b ) gated, isotype-switched B cells analysed for reactivity against NP antigen (NP + , IgG1 + ). ( c ) NP + IgG1 + B cells were further fractionated into germinal center (GC) and memory compartments on the basis of CD38 expression. ( d ) Absolute numbers of NP + IgG1 + B cells per spleen. ( e ) Frozen sections of spleens 14 days post immunization stained with IgD (green) to identify B-cell follicles and GL-7 (red) to identify GC. Scale bars, 400 μm. White arrows indicate GC structures. Data are mean±s.e.m. of five mice per group. Data are representative of three independent experiments. Significance of differences were determined using two-tailed unpaired t -tests. * P <0.05. Full size image In vitro , vorinostat had similar effects to panobinostat on B-cell survival, proliferation and differentiation. As vorinostat is used clinically for a range of diseases [18] , we thought it pertinent to determine whether similar immunosuppressive effects were observed. As with panobinostat, the production of B220 + IgD lo NP + IgG1 + B cells was reduced after vorinostat treatment ( Supplementary Fig. 11a–d ) and GC formation in spleens severely disrupted ( Supplementary Fig. 11e ). These results conclusively demonstrate that treatment with compounds that target multiple HDACs significantly impedes functional primary antibody responses. Humoral memory is not affected by HDACi treatment We reasoned that an important clinical question for cancer patients receiving HDACi therapy, and a potential hurdle in their use for B-cell-driven autoimmune disease, is the possible impact on memory B cells that may have been generated many years earlier. In a clinical setting, this would manifest post cessation of HDACi therapy, so we measured the effect of panobinostat on memory-recall responses of NP–KLH-immunized mice. C57BL/6 mice immunized with adjuvanted NP–KLH were left for 40 days, so memory B cells had been generated. These mice were then treated with panobinostat or vehicle. A striking depletion of the naive B-cell population was observed following panonobinostat treatment ( Supplementary Fig. 12a ). Following panobinostat-induced B-cell depletion, mice were rested for 12 days before being re-challenged with NP–KLH in the absence of adjuvant. Surprisingly, panobinostat-treated mice generated a robust memory response with no difference in the proportion of B220 + IgD lo B cells ( Fig. 6a ), or the proportion of NP + IgG1 + antigen-specific cells within this population ( Fig. 6b ) being observed. NP + IgG1 + cells were validated as genuine memory cells via expression of CD38 ( Fig. 6c and Supplementary Fig. 8b ) and by the significant increase in the number of NP-responsive B cells after immunization ( Supplementary Fig. 12b ). Importantly, treatment with panobinostat did not affect the numbers of these antigen-specific memory cells after boosting illustrating the memory response to be intact ( Fig. 6d and Supplementary Fig. 12b ). Similarly, vorinostat treatment had no effect on the ability to generate a robust memory response ( Supplementary Fig. 13 ). 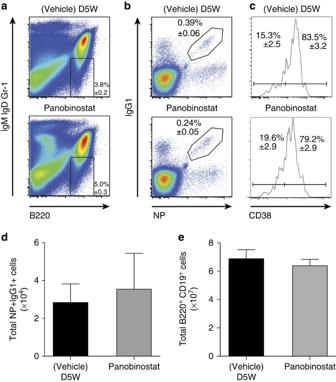Figure 6: Memory antibody responses are not affected by panobinostat treatment. C57BL/6 mice were immunized with NP–KLH and rested for 40 days. Cohorts were then treated with vehicle or panobinostat for 1 week, rested for 12 days, and then re-challenged with NP–KLH and analysed 5 days later to assess memory responses. (a) Flow cytometric identification of isotype-switched splenic B cells (GR-1−, IgM−, IgD−, B220+). (b) Gated, isotype-switched B cells were analysed for NP reactivity (NP+IgG1+) and (c) memory cells identified on the basis of CD38 expression. Absolute numbers of (d) NP+IgG1+B cells and (e) B220+CD19+B cells per spleen. Data are mean±s.e.m. of four mice per group from two independent experiments. Significance of differences were determined using two-tailed unpairedt-tests. Figure 6: Memory antibody responses are not affected by panobinostat treatment. C57BL/6 mice were immunized with NP–KLH and rested for 40 days. Cohorts were then treated with vehicle or panobinostat for 1 week, rested for 12 days, and then re-challenged with NP–KLH and analysed 5 days later to assess memory responses. ( a ) Flow cytometric identification of isotype-switched splenic B cells (GR-1 − , IgM − , IgD − , B220 + ). ( b ) Gated, isotype-switched B cells were analysed for NP reactivity (NP + IgG1 + ) and ( c ) memory cells identified on the basis of CD38 expression. Absolute numbers of ( d ) NP + IgG1 + B cells and ( e ) B220 + CD19 + B cells per spleen. Data are mean±s.e.m. of four mice per group from two independent experiments. Significance of differences were determined using two-tailed unpaired t -tests. Full size image To determine whether panobinostat or vorinostat would affect subsequent regeneration of naive B-cell populations from haematopoietic stem cells (HSC) or more differentiated B-cell progenitors, we measured the number of CD19 + B220 + B cells in the spleens of mice 17 days after termination of HDACi treatment. Interestingly, there was no significant difference in the total number of CD19 + B220 + B cells in spleens of mice following termination of panobinostat ( Fig. 6e ) or vorinostat treatment ( Supplementary Fig. 13e ), indicating that homeostatic B lymphopoiesis was intact and suggesting that B-lineage progenitors remained viable and functional after HDACi treatment. HDACi are potent epigenetic regulators used effectively to treat haematological malignancies [18] . Despite their successful use as anticancer agents and potential as immunomodulatory compounds [25] , [26] , [27] , [28] , [36] , [46] , they have not been used clinically for modulation of the immune system. Here, we demonstrate that B-cell function is particularly sensitive to modulation with HDACi. In vitro , HDACi are capable of altering diverse aspects of the B-cell response in an HDAC-class-dependent manner that is maintained for both T-cell-dependent or -independent activation. The pan-HDACi vorinostat and panobinostat modified survival, proliferation and differentiation, whereas the class-I-selective HDACi romidepsin predominantly reduced B-cell survival, leaving proliferation and differentiation intact. These selective differences are not unexpected, as romidepsin has been demonstrated to have a restricted set of targets when compared to pan-HDACi [47] and this specificity manifests at both the molecular [48] and functional level [49] . The broad effect of panobinostat and vorinostat on B cells in vitro , coupled with the strong effect on multiple myeloma plasma cells [19] , indicated that these compounds could have potential applications targeting self-reactive B-cell populations in vivo . Panobinostat stands as a particularly exciting therapeutic option as it is capable of modifying multiple aspects of the B-cell response at low nanomolar concentrations while leaving CD8 + T-cell responses unaffected in vitro . These properties of panobinostat provided the intriguing potential to treat B-cell-mediated autoimmune disease without concurrent risk of T-cell immunosuppression. This potential could be realized at much lower doses than are required for anti-neoplastic effects, conveying greater tolerability. Similarly, results in graft versus host studies have demonstrated that vorinostat has a strong immunosuppressive T-cell effect, in contrast to panobinostat [36] . The ability of panobinostat to eliminate plasma cells in autoimmune mouse models with severe genetic abnormalities also suggests that they may be effective in the human setting, where self-reactive clones are more rare, and their generation is dependent on a combination of multiple genetic susceptibility loci [50] . The ability to target B cells stimulated in both a T-independent and T-dependent manner suggests that HDACi therapy might allow targeting of autoreactive B cells that are generated by either polyclonal activation or as a consequence of a GC-related event. A similar rationale using anticancer agents such as the B-cell-depleting antibody rituximab (anti-CD20) to dampen the antibody response has been proposed for treating autoimmunity. However, clinical trials with these therapies has been disappointing, possibly because they are less effective at targeting plasma cells; moreover, they can cause long-term B-cell immunosuppression [51] , [52] . Thus, the potent effect of panobinostat on the B-cell lineage (including plasma cells) stands as an exciting potential novel therapeutic for treatment of SLE. Furthermore, the rapid replacement of naive B cells at cessation of treatment suggests long-term B-cell immunosuppression through depletion of lymphoid progenitor cells might also be avoided. A potential danger of using HDACi as an immunomodulatory therapeutic is the possible effects on bystander populations. Our results demonstrate that T cells are considerably less sensitive than B cells to panobinostat treatment in vitro and in vivo, even after 6 weeks of continued administration. An additional, subset-specific effect is that unlike naive B cells and autoreactive plasma cells, memory B cells were insensitive to panobinostat treatment in vivo . Furthermore, the recovery of normal B-cell numbers 17 days after cessation of HDACi treatment suggests that the function of HSC and B-cell progenitor populations might be potentially protected Long-term. Although the reasons for the observed differences in sensitivity to panobinostat are unclear, perhaps the distinct transcriptional responses of lymphocyte subsets, progenitor populations and malignant cells instill particular resistance or sensitivity to HDACi. Indeed, we have observed that isogenic matched normal and tumour cells display subtle differences in transcriptional responses to HDACi resulting in profound differential biological responses [53] . In reference to the differential targeting of naive B cells and memory B cells, the finding that B cells have a stage-specific dependence on anti-apoptotic molecules during the generation of primary and memory B-cell responses [54] , combined with selective targeting of these genes by HDACi supports this rationale. Although deciphering the molecular events that underpin the differential effects of structurally diverse HDACi on normal and pathogenic lymphocytes is of interest, the expanded clinical application of these HDACi in the oncology setting without such mechanistic knowledge, supports in our opinion the argument that HDACi should similarly be tested in humans for the treatment of certain autoimmune diseases. Our results provide rationale for conducting similar studies using HDACi that recognize a more restricted range of targets. More specific HDACi might have the potential to refine immune cell subsets targeting an even smaller set of candidates. Data from our in vitro studies with vorinostat also suggest the potential to modify T-cell responses if the HDAC associated with their function can be identified. We believe that cross referencing both functional and gene expression studies using inhibitors with intersecting HDAC specificity has the potential to provide significant insight into the epigenetic mechanisms involved in the regulation of autoreactive and protective immune responses. Our results suggest that HDACi such as panobinostat may have important clinical applications in the treatment of antibody-driven autoimmune conditions. As the reported side effects of long-term HDACi treatment in cancer patients have been demonstrated to be manageable [18] , [55] , and panobinostat treatment in multiple myeloma patients has been well tolerated with significant disease benefit [39] , this suggests that if the short-term immunosuppression can be managed effectively, an HDACi-based therapy could be well tolerated in autoimmune disease patients. At the low doses anticipated in the treatment of autoimmune disease, potential B-cell-dependent immune suppression could be treated with treatment interruption or dose reduction. In addition, our results demonstrate that immunosuppression induced by HDACi treatment only affects the generation of new or existing antibody responses. This is clinically relevant as it suggests that prophylactic vaccinations should be considered before embarking on a course of HDACi therapy for autoimmune disease or cancer treatment, but equally that protective immunity may be retained. Importantly, the production of new B cells by the haematopoietic compartment to replace those targeted by treatment, and the function of circulating memory B cells, is intact. These results have exciting implications for the refinement of HDACi treatment in the clinic for both autoimmune disease and cancer patients. Mice and immunization protocols The animal experiments in this study were performed as approved by the animal experimentation ethics committee of the Peter MacCallum Cancer Centre, Victoria, Australia. Male and female MRL /lpr mice [56] either 7 weeks of age for germinal centre experiments or >12 weeks of age for autoimmune pathology experiments were purchased from the Walter and Eliza Hall Institute (Kew, Victoria, Australia). Male and female Lyn −/− mice aged 5 months were on a C57BL/6 background and have been described in refs 42 , 57 . For immunization experiments, 8–14-week-old male or female C57BL/6 mice received a single intraperitoneal injection of 50 μg nitrophenyl coupled to keyhole limpet haemocyanin (NP–KLH) at a ratio of 21:1 and precipitated onto alum, prepared as described [58] . For memory responses, mice received a second dose of 10 μg of NP–KLH in PBS >40 days after the initial immunization. To determine immune response to NP immunization, single-cell suspensions were stained as described [59] using antibodies to the following surface molecules: CD38 (NIMR-5), B220 (RA3-6B2), IgM (331.12), IgD (11-26C), Gr-1 (RB6-8C5), CD138 (281.2), IgG1 (X56;BD Pharmingen), GL-7 (ref. 58 ), CD19 (1D3; BD Pharmingen). NP binding was detected as described [59] . Cells were analysed on an LSRII or Canto (BD Biosciences). Cell culture of mouse lymphocytes All lymphocytes were isolated from 8- to 16-week-old C57BL/6 mice. B cells were prepared, CFSE labelled and cultured as described [30] , [60] . Cell numbers were determined by reference to FACS calibration beads as described [29] , [31] . B cells were typically >95% B220 + , CD19 + , IgM + , IgD + as determined by flow cytometry. Stimuli were added as follows: lipopolysaccharide derived from Salmonella typhosa (LPS, Sigma-Aldrich, St. Louis, MO, USA) and αCD40 antibody (clone FGK4.5, WEHI) were at used at 20 μg ml −1 . IL-4 (R&D Systems, Minneapolis, MN, USA) was added at 20 ng ml −1 . For in vitro differentiation studies, B cells were stained for expression of CD138 (clone 281-2, BD Pharmingen). For analysis of CD8 T-cell responses, CD62L Hi CD8 + T cells were prepared from lymph nodes using MACS negative selection kits (Miltenyi Biotec, Auburn, CA, USA). T cells were activated with 10 μg ml −1 plate-bound αCD3 clone 145-2C11 (eBioscience, San Diego, CA, USA) in the presence of 100 U ml −1 saturating IL-2 (R&D Systems, Minneapolis, MN, USA). T cells were CFSE labelled and the analysis of cell survival and proliferation performed as described [29] . HDAC inhibitors Panobinostat was kindly provided by Novartis (Basel, Switzerland), vorinostat by Merck (Boston, MA, USA) and romidepsin was obtained from Celgene (Summit, USA). Panobinostat and romidepsin were diluted in 5% dextrose water (D5W). Vorinostat was diluted in DMSO. For in vitro experiments, concentrations were used as indicated in figures. Vehicle controls correspond to the highest proportion of vehicle used in each experiment. HDACi were administered in vivo by intraperitoneal injection using the dosing regime as follows: NP–KLH immunization studies, both primary and secondary immunization: 10 mg kg −1 panobinostat and 200 mg kg −1 vorinostat days 1–3, rested day 4, then days 5–7; treatment of autoimmune mice: 10 mg kg −1 panobinostat day 1–15 followed by 5 mg kg −1 days 16–41; 200 mg kg −1 vorinostat day 1–3, 150 mg kg −1 day 5–41. Treatment was halted for 1 or 2 days per week to avoid toxicity. For all in vivo experimentation (NP–KLH immunization and treatment of autoimmune mice), mice were monitored and subsets analysed by a separate researcher masked to treatment group allocation. Immunohistochemistry Immunohistochemistry was performed as described [58] . Antibodies used were unlabelled rat anti-GL-7 (ref. 58 ) at a final concentration of 10 μg ml −1 and biotinylated anti-IgD (Southern Biotech, Birmingham, AL, USA) at a final concentration of 5 μg ml −1 . For NP–KLH immunization studies, the following secondary antibodies were used: anti-rat-Alexa-488 or 546 and streptavidin-488 or 546, (Molecular Probes) all at a dilution of 1:100. For MRL/ lpr studies, GL-7 was detected with anti-rat HRP (Invitrogen, final dilution 1:100) and biotinylated anti-IgD with streptavidin–alkaline phosphatase (final dilution 1:100). Sections were imaged using a Fluoview FV1000 confocal microscope (Olympus, Japan) with a 12.9 mW 488 nm multi-ion Argon laser, 1 mW 543 nm multi-ion green HeNe laser and 11 mW 633 nm red HeNe laser. Sections from MRL/lpr mice were imaged using a Zeiss Axioplan 2 (Zeiss, Oberkochen, Germany). Analysis of autoimmune mice Blood was isolated from the retro-orbital sinus of mice at the indicated time points. Immune subsets were quantified per 50 μl aliquot of peripheral blood. Red blood cells were lysed and stained for subsets using antibodies against CD4, CD8, CD62L, B220, CD19, CD138. Total cell numbers were determined by reference to a known number of calibration beads as described [29] . Serum for antinuclear antibody analysis was incubated with pre-coated nuclear antigen plates (Cat#MK200, The Binding Site, Birmingham, AL, USA), and murine Ig detected with goat anti-mouse Ig (H+L)-HRP (cat#1010-05 Southern Biotech Associates). Renal pathology was graded according to standard methods for the assessment of diffuse proliferative lupus nephritis on haematoxylin and eosin-stained sections [61] . Severity scores were assigned by the consensus opinion of two pathologists (J.S. and I.S.) who were double-masked to treatment group allocations. The scoring system for glomerular and interstitial inflammatory and proliferative changes was performed as previously described [25] . Briefly, a score of 0–3 was assigned to each of the following: glomerular inflammation, proliferation, crescent formation, necrosis and interstitial/hilar infiltrate. Scores for crescent formation and necrosis were doubled before adding to yield a composite total (with a maximum possible aggregate of 21). Method for ENA testing ENA in sera were measured using the FIDIS Connective Profile MX 117 kit (Theradiag) according to manufacturer’s instructions, except a PE-conjugated polyclonal anti-mouse IgG F(ab’)2 secondary antibody (eBioscience, cat. no. 12-4010) was used to detect binding of mouse autoantibodies and fluorescence was measured using a BD FACSCanto II (BD Bioscience). Statistical analyses Average values are reported as the mean±s.e.m. Unpaired t- tests and ANOVA were performed using Prism 6.0 (GraphPad Software, Inc.) to determine the statistical significance of the data. How to cite this article: Waibel, M. et al. Manipulation of B-cell responses with histone deacetylase inhibitors. Nat. Commun. 6:6838 doi: 10.1038/ncomms7838 (2015).